Ultra-high-energy cosmic ray acceleration in engine-driven relativistic supernovae The origin of ultra-high-energy cosmic rays (UHECRs) remains an enigma. They offer a window to new physics, including tests of physical laws at energies unattainable by terrestrial accelerators. They must be accelerated locally, otherwise, background radiations would severely suppress the flux of protons and nuclei, at energies above the Greisen–Zatsepin–Kuzmin (GZK) limit. Nearby, gamma ray bursts (GRBs), hypernovae, active galactic nuclei and their flares have all been suggested and debated as possible sources. A local sub-population of type Ibc supernovae (SNe) with mildly relativistic outflows have been detected as sub-energetic GRBs, X-ray flashes and recently as radio afterglows without detected GRB counterparts. Here, we measure the size-magnetic field evolution, baryon loading and energetics, using the observed radio spectra of SN 2009bb. We place such engine-driven SNe above the Hillas line and establish that they can readily explain the post-GZK UHECRs. The highest energy cosmic rays pack such a large amount of energy and have such a low flux [1] that direct detection by satellite-borne instruments is infeasible, allowing them to be detected [2] only by cosmic ray air showers [3] . Ultra-high-energy cosmic rays (UHECRs) beyond the Greisen–Zatsepin–Kuzmin (GZK) limit [4] , [5] have been invoked to propose tests of known physical laws and symmetries [6] . Understanding their origin is a crucial step in using them as probes of new physics. But, the sources of the highest energy cosmic rays pose an intriguing problem, as the magnetic rigidity of these particles are such that the magnetic fields in our galaxy are neither strong enough to contain them nor bend them sufficiently [2] . Yet, among the UHECRs, which have been detected until now, no concentration has been found towards the Milky Way. Hence, it is anticipated that their sources are extragalactic. However, UHECR protons with energies above 60 EeV can interact with a significant fraction of cosmic microwave background (CMB) photons via the Δ resonance. The cross-section of this interaction is such that only local extragalactic cosmic ray sources (within 200 Mpc of the Earth) can contribute significantly to the flux of UHECRs above the so-called GZK limit [4] , [5] , [7] . Many sources are required by observations of UHECRs until now, to explain the 61 cosmic rays detected [1] with energies above the GZK limit. As particles of such high energy could not have travelled to the Earth from cosmological distances, unless Lorentz invariance breaks down at these energies [6] , they encourage the search for potential cosmic ray accelerators in the local Universe. Active galactic nuclei (AGNs) have been considered [1] as UHECR sources. But according to Farrar et al . [8] , most of them are not luminous enough, leaving proposed very intense, short duration AGN flares, which are yet to be observed, as possible sources [8] . Gamma ray bursts (GRBs) are also considered as possible sources [9] , [10] , [11] , but most of them occur beyond the GZK horizon [12] and cannot contribute significantly to the local flux beyond the GZK limit [8] . Hypernovae have also been suggested as sources, in which particles are boosted to successively higher energies in an ejecta profile extending up to mildly relativistic velocities [13] , [14] . However, they require excessive explosion energy and fail to reproduce the flat injection spectrum of UHECRs (see Supplementary Discussion for some of the proposed sources). Soon after their suggestion that supernovae (SNe) come from collapse of a normal star to a neutron star, Baade and Zwicky [15] went on to suggest that SNe may be the source of cosmic rays as well. Since then, SNe and supernova remnants (SNR) have been studied as sources of high-energy cosmic rays. However, ordinary SNe and their remnants cannot produce UHECRs because of two fundamental limitations. First, they lie well below the line representing the combination of size and magnetic field required to confine and accelerate iron nuclei with energies of 60 EeV, in the so-called Hillas diagram [16] ( Fig. 1 ). The second, even more restrictive, condition obviously not fulfilled by ordinary SNe is because ordinary SNe have β /Γ ∼ 0.05 ( β≡v/c and where v is the speed of the blast wave and c is the speed of light in vacuum), which restricts the highest energy cosmic rays accelerated in ordinary SNe to well below the GZK limit. 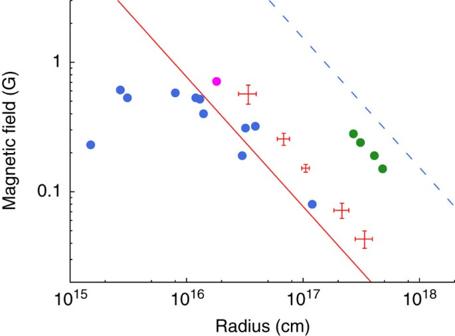Figure 1: Hillas diagram. Mildly relativistic sources (β/Γ∼1) must lie above the solid red line, to be able to accelerate iron nuclei to 60 EeV by diffusive shock acceleration31, according toEZ≲βeZBR/Γ(ref.40). In comparison, non-relativistic SNe (β/Γ∼0.05) must lie above the dashed blue line to reach the same energies. Radius and magnetic field of SN 2009bb (red crosses, at 5 epochs, determined here from radio observations with VLA and GMRT assuming equipartition) and XRF 060218 (ref.18; magenta ball) lie above the solid red line. Other20radio SNe with SSA fits are plotted as blue balls. Only the SN 1993J magnetic fields are obtained without assuming equipartition36. Note that all of the observed non-relativistic SNe (blue balls) including SN 1993J (green balls) lie below the dashed blue line and are unable to produce UHECRs unlike the mildly relativistic SN 2009bb and XRF 060218, which lie above the red line. Sizes of crosses are twice the statistical standard errors, sizes of balls are bigger than the standard errors. Figure 1: Hillas diagram. Mildly relativistic sources ( β /Γ ∼ 1) must lie above the solid red line, to be able to accelerate iron nuclei to 60 EeV by diffusive shock acceleration [31] , according to E Z ≲ βeZBR/Γ (ref. 40 ). In comparison, non-relativistic SNe ( β /Γ ∼ 0.05) must lie above the dashed blue line to reach the same energies. Radius and magnetic field of SN 2009bb (red crosses, at 5 epochs, determined here from radio observations with VLA and GMRT assuming equipartition) and XRF 060218 (ref. 18 ; magenta ball) lie above the solid red line. Other [20] radio SNe with SSA fits are plotted as blue balls. Only the SN 1993J magnetic fields are obtained without assuming equipartition [36] . Note that all of the observed non-relativistic SNe (blue balls) including SN 1993J (green balls) lie below the dashed blue line and are unable to produce UHECRs unlike the mildly relativistic SN 2009bb and XRF 060218, which lie above the red line. Sizes of crosses are twice the statistical standard errors, sizes of balls are bigger than the standard errors. Full size image Until recently, SNe with relativistic ejecta have been spotted exclusively through long GRBs associated with them like GRB 980425 (ref. 17 ) or its twin GRB 031203. The discovery of XRF 060218 (ref. 18 ) associated with SN 2006aj showed that mildly relativistic SNe are 100 times less energetic, but 1,000 times more common (in their isotropic equivalent rate, which is relevant for UHECRs actually reaching the observer) than classical GRBs [18] . Radio follow-up of SNe Ibc have now revealed the presence of an engine-driven outflow from SN 2009bb (ref. 19 ), without a detected GRB. The mildly relativistic SNe, detected either using X-ray flashes (XRFs) or radio afterglows, a subset of SNe Ibc are far more abundant at low redshifts required for the UHECR sources, than the classical GRBs. Moreover, given their mildly relativistic nature, they have the most favourable combination of β /Γ ∼ 1, unlike both non-relativistic SNe and ultra-relativistic classical long GRBs. In this work, we have measured the size-magnetic field evolution of the prototypical SN 2009bb. We place such engine-driven SNe above the Hillas line and demonstrate that they may accelerate cosmic rays to beyond the GZK threshold. Coupled with the rates and energetics of such events, discussed in this work, we establish that they may readily explain the post-GZK UHECRs. Radius-magnetic field evolution To derive the highest energy, up to which these relativistic SNe can accelerate cosmic rays (see Fig. 1 ), we have to determine the evolution of the size and the magnetic field in the blast wave. It has been demonstrated that a Synchrotron Self-Absorption (SSA) model fits the initial radio spectrum of SN 2009bb rather well [19] , with a low frequency turnover defining the spectral peak shifting to lower frequency with time, characteristic of the expansion of the shocked region that powers the radio emission. This allows us to measure the evolution of the radii and magnetic fields from Very Large Array (VLA) and Giant Metrewave Radio Telescope (GMRT) data at 5 epochs, plotted on the Hillas diagram ( Fig. 1 ). With a robust set of assumptions for the electron energy distribution and magnetic fields [20] , the radius of the forward shock wave at the time of the SSA peak can be written as [20] where α = ɛ e / ɛ B is the ratio of relativistic electron energy density to magnetic energy density, f is the fraction of the spherical volume occupied by the radio emitting region, F op is the observed peak flux, and D is the distance. Using the same variables, the magnetic field is given by The radio spectrum of SN 2009bb at all epochs from discovery paper (Fig. 2 of ref. 19 ) and this work, as obtained from observations using the VLA and the GMRT, is well fit by the SSA model, giving us a rare opportunity to explicitly measure the size and magnetic field of a candidate accelerator, instead of indirect arguments connecting luminosity with the Poynting flux. This clearly demonstrates that SN 2009bb and XRF 060218 can both confine UHECRs and accelerate them to highest energies seen experimentally. At the time of the earliest radio observations [19] with its fortunate combination of β /Γ ∼ 1, SN 2009bb could have accelerated nuclei of atomic number Z to an energy of ∼ 6.5 × Z EeV. For example, the source could have accelerated protons, neon and iron nuclei to 6.4, 64 and 166 EeV, respectively. In this scheme, the highest energy particles are likely to be nuclei heavier than protons, consistent with the latest results indicating an increasing average rest mass of primary UHECRs with energy [21] . Therefore, our results support the claimed preference of heavier UHECRs at the highest energies of the Auger collaboration, although this claim is disputed by another experiment [22] . Rates of engine-driven SNe To estimate whether there are enough relativistic SNe to explain the target objects associated with the ∼ 60 detected UHECRs, we require the rate of such transients. SNe Ibc occur at a rate [23] , [24] of ∼ 1.7 × 10 4 Gpc −3 per year. The fraction of Ibc, which have relativistic outflows, is still a somewhat uncertain number, estimated [19] to be around ∼ 0.7%. Hence, the rate of SN 2009bb-like mildly relativistic SNe is ∼ 1.2 × 10 −7 Mpc −3 per year, which is comparable to the rate of mildly relativistic SNe detected as sub-energetic GRBs or XRFs of ∼ 2.3 × 10 −7 Mpc −3 per year. This gives us ∼ 4 (or 0.5) such objects within a distance of 200 (or 100) Mpc every year. As SN 2009bb is still a unique object, only a systematic radio survey can establish their cosmic rate and statistical properties. However, cosmic rays of different energies have different travel delays due to deflections by magnetic fields. For a conservative mean delay [8] of 〈 τ delay 〉≈ 10 5 years, we may receive cosmic rays from any of 4 (or 0.5) × 10 5 possible sources at any point in time. Given the situation, in which a direct association between a detected UHECR and its source is unlikely [25] , the literature in the subject has focused on the constraints [16] , [26] placed on plausible sources. We have shown in our work that indeed this new class of objects satisfy all these constraints. Nuclei are also subject to photo-disintegration by interaction with Lorentz boosted CMB photons and can travel up to a distance of ∼ 100 Mpc (see Methods ), smaller than but comparable to the GZK horizon. So, the local rate of mildly relativistic SNe is high enough to provide enough ( ≫ 60) independent sources of cosmic rays with energies above the GZK limit. The value of 〈 τ delay 〉 also implies that it will not be possible to detect UHECRs from a known relativistic SN, such as SN 2009bb, within human timescales. However, high-energy neutrinos from photo-hadron interaction at the acceleration site may be a prime focus of future attempts at detecting these sources with neutrino observatories like the IceCube (see Methods ). Energy injection The required energy injection rate per logarithmic interval in UHECRs [9] , [27] is Γ inj =(0.7–20) × 10 44 erg Mpc −3 per year. Given the volumetric rate of mildly relativistic SNe in the local universe, if all the energy injected into UHECRs is provided by local mildly relativistic SNe, then each of them has to put in around E SN =(0.3–9) × 10 51 ergs of energy, which is comparable to the kinetic energy in even a normal SN and can easily be supplied by a collapsar model [28] . The minimum energy in the relativistic outflow of SN 2009bb, required to explain the radio emission alone, was found [19] to be E eq ≈ 10 49 ergs at 20 days. Moreover, the mildly relativistic outflow of SN 2009bb has been undergoing almost free expansion for ∼ 1 year. Our measurements of this expansion allows us to show (see Energy Budget in SN 2009bb ) that this relativistic outflow, without a detected GRB, is significantly baryon loaded and the energy carried by the relativistic baryons is E Baryons ≳ 3.3 × 10 51 ergs. Energy budget in SN 2009bb The radius evolution of SN 2009bb, as inferred from our radio observations ( Table 1 ), is consistent with nearly free expansion. This can only be explained if the mass of the relativistic ejecta is still much larger than the swept up mass. The computed Lorentz factor has barely decreased from 1.32 to 1.23 between days 20 and 222 post-explosion. Using the model for collisional slow down of the ejecta, we modify equation 115 of ref. 29 , to give where m ( R 1 ) and m ( R 2 ) are the swept up mass at the two respective epochs. We have neglected radiative losses, as they are unlikely to be important for protons in the time range of interest. Moreover, radiative losses would only help increase our initial energy budget. Performing the integral numerically (see ref. 30 for an analytic solution) from γ 1 to γ 2 , the Lorentz factors at the two epochs and substituting for m ( R ) using the progenitor mass loss rate [19] , we solve for the ejecta mass to get M 0 ≈1.4×10 −3 M ⊙ . Most of the mass in the relativistic outflow is due to baryons. The energy associated with these relativistic protons and nuclei is found to be E Baryons ≳ 3.3 × 10 51 ergs. Compared with this blast-wave calorimetric value, the equipartition energy in the electrons and magnetic fields determined from SSA fit to the radio spectrum was reported [19] to be E eq ≈ 1.3 × 10 49 ergs. This gives the electrons only a fraction of the energy in the relativistic baryons. If E Baryons is distributed equally over ten decades in energy, it can account for ∼ 0.33 × 10 51 ergs of energy in UHECRs per logarithmic energy interval. Given the rate of relativistic SNe in the local universe, this is consistent with the volumetric energy injection rate for UHECRs. Table 1 Radius-magnetic field evolution. Full size table Observational signatures If a relativistic outflow carries similar energies in protons, electrons and magnetic fields, the radiative cooling of the electrons will lead to an X-ray transient [26] . In our model, the acceleration occurs in the forward shock produced by the engine-driven relativistic ejecta, characterized by a single bulk Lorentz factor. Protons and nuclei in such a collisionless shock show a flat spectrum of UHECRs [31] , consistent with the extragalactic component of the cosmic ray spectrum [27] . Our radio observations of SN 2009bb constrain the energy carried by the radiating electrons [19] and the energy of the relativistic baryons powering the almost free expansion for ∼ 1 year until now. These observations indicate a spectral index of ≈1 in the optically thin part of the radio spectrum [19] . This implies a power-law distribution of relativistic electrons, with an energy index between p ≈ (2–3), depending on the relative positions of the breaks in its spectra [29] . The observed rate of relativistic SNe in the local universe is consistent with the required rate of X-ray [26] and radio (see Methods ) transients accompanying the UHECR accelerators. Rate of radio transients The required rate of radio transients, which can supply the observed Γ inj is given by . Assuming that the electrons and magnetic fields together have a fraction ɛ of the energy of the relativistic protons (which is assumed to be divided equally into ∼ 10 logarithmic bins, assuming p ≈2 for the protons), we compute the minimum required rate of such transients with peak radio luminosity L op , which remain mildly relativistic at least until the SSA peak frequency drops to v , as Here, is the ratio between the observed angular radius and the one obtained by assuming equipartition between electrons and magnetic fields [17] . This criterion works for an electron energy index between p =2 (with the cooling break shifted below the SSA peak) to p =3 (with the cooling break above the observed radio frequencies), so as to explain the observed spectral index of ≈1 in the optically thin part of the radio spectrum. Here, equation (4) is the radio analogue of equation 2.5 of ref. 26 (which is for X-ray transients). Hence, the observed rate of relativistic SNe can easily explain the energy injection rate. Proposed survey parameters The prototypical mildly relativistic SN 2009bb has been discovered [19] in a dedicated radio follow-up of type Ibc SNe. To firmly establish the rate of occurrence of such relativistic SNe in the local universe, a systematic large area radio survey is required. Here, we estimate the maximum energy to which relativistic SNe can accelerate nuclei of charge Z e from E Z ≲ Z e BR as β /Γ ∼ 1 for mildly relativistic outflows. Substituting the expressions for the radius (equation (1)) and magnetic field (equation 2)) we have which is independent of the observed SSA peak frequency v . Further, assuming that R ∼ Γ β ct and we get the time to reach the synchrotron peak is Hence, relativistic SNe will have faster rise times than non-relativist radio transients, allowing them to be easily identified for multi-frequency follow-up with targeted observations. These considerations determine the cadence and sensitivity of the proposed radio survey as mentioned in the main text. It has been found that the arrival direction of the Auger events correlate well with the locations of nearby AGNs [1] , this suggests that they come from either AGNs or objects with similar spatial distribution as AGNs. Note that the correlation appears weaker in subsequent data [32] and the HiRes events [33] do not show such a correlation. Furthermore, UHECRs correlate well [34] with the locations of neutral hydrogen (HI)-rich galaxies from the HI Parkes All Sky Survey. Our proposal relies on the acceleration of UHECRs in the mildly relativistic outflow from a subset of SNe Ibc, for which we have determined the size and magnetic field evolution using our radio observations, rather than hypothetical magnetars, with as yet unknown magnetic fields, supposedly formed during sub-energetic GRBs [34] considered in that work. SNe Ibc occur mostly in gas-rich star-forming spirals. In particular, the 21 cm flux of NGC3278 (hosting SN 2009bb) obtained from the HyperLeda database [35] amounts to ∼ 1.9 × 10 9 M ⊙ of HI. Hence, the observed correlation of UHECR arrival directions with HI-selected galaxies [34] is consistent with our hypothesis. In this article, we have shown that the newly established subset of nearby SNe Ibc, with engine-driven mildly relativistic outflows detected as sub-energetic GRBs, XRFs or solely via their strong radio emission, can be a source of UHECRs with energies beyond the GZK limit. Our study demonstrates for the first time, a new class of objects, which satisfy the constraints that any proposed accelerator of UHECRs has to satisfy. If SN 2009bb is characteristic of this newly discovered class, a radio survey to detect all such events should be undertaken. As an example, an all sky radio survey at v =1 GHz with a sensitivity of 1 mJy and cadence of 2 months, can detect all such transient sources, which can accelerate Neon nuclei to 60 EeV, within 200 Mpc of the Earth ( ∼ 4 per year). Such a survey will also detect radio emission from ordinary SNe and non-relativistic transients. However, their faster rise to peak will easily separate out the relativistic SNe for multi-frequency follow-up. Equipartition As already stated, non-relativistic SN have sizes and magnetic fields which are characteristically inadequate to accelerate charged particles to the highest energies. However, the inferred magnetic fields are based mostly on equipartition arguments. The only young SN, in which the magnetic field was determined independent of the equipartition assumption, was SN 1993J (this was, however, a type IIb SN, unlike the type Ibc's being considered here). However, the magnetic field determined using a synchrotron cooling break was found to be approximately nine times larger than the equipartition value [36] . This only helps by placing the SN 1993J much closer to the Hillas line (but still below it) due to enhanced BR product. The energy requirement to explain the radio emission has a minimum [17] at the assumed equipartition factor of α =1. In the absence of an independent measurement of the magnetic field, as in SN 1993J (ref. 36 ), Very Long Base Interferometry of the outflow can constrain the deviation from equipartition using equation (1). However, because of the very slow dependence of the radius on α , even for a slight deviation from equipartition in SN 2009bb, it can easily inflate the energy in the radio emitting plasma. In the case of SN 2009bb, even a more conservative assumption of equipartition, aided by its demonstrated mildly relativistic outflow enables it to be in a class of SN, which can readily account for possible accelerators of UHECRs. Rate of X-ray transients The number density of XRFs associated with UHECR accelerators has been prescribed [26] assuming that the accelerated electrons have the same initial power-law index for their energy spectrum as the protons, and that they lose all their energy radiatively. Using the values of the physical parameters, motivated by SN2009bb, the number density of active XRFs with a luminosity ≳ vL v is then given by recasting equation 2.5 of ref. 26 to give SN 2009bb was observed with the Chandra ACIS-S instrument, at age 31 days, in the energy range 0.3–10 keV. It had an X-ray luminosity [19] of L X = 4.4±0.9× 10 39 erg s −1 . This luminosity and the rate of the relativistic SNe, considered in this work, together can account for the UHECR flux, if they remain active accelerators for Δ t of order ∼ 1 year. This is consistent with our radio observations, which confirm that the BR product remains above the threshold throughout the ∼ 1 year of observation (see Table 1 ). Propagation and survival of nuclei In the particle acceleration scheme outlined in this work, the highest energy particles are likely to be nuclei rather than protons. This is borne out by the latest Auger data, which favours an increasing average rest mass of primary cosmic ray particles at the highest energies [21] . As for protons, the flux of ultra-high-energy nuclei are also suppressed over cosmological distances via interaction with background radiations. CMB photons appear has high-energy γ -rays when Lorentz boosted into the rest frames of ultra-high-energy protons or nuclei. Protons above ∼ 60 EeV, interact with CMB photons via the Δ resonance or and give rise to the GZK limit [4] , [5] . Similarly, ultra-high-energy nuclei can be photo-disintegrated by Lorentz boosted cosmic infrared background photons interacting mainly via giant dipole resonances. The distance over which this effect suppresses the flux of ultra-high-energy nuclei is a function of the nuclear species and its energy. Detailed calculations [37] using updated photo-disintegration cross-sections indicate that the energy loss lengths for 100 EeV intermediate mass nuclei such as Ne, Si and Ca are around ∼ 100 Mpc. As discussed in the main text, relativistic SNe can provide enough number of UHECR sources within this distance, to be consistent with observation of independent arrival directions for the UHECRs. High-energy particle detection UHECRs from the same source but with different energies will travel by different trajectories due to deflections by magnetic fields [9] . For current estimates of the average intergalactic magnetic field, the mean delay in the arrival time of UHECRs, when compared with photons is found [8] 〈 τ delay 〉≈ 10 5 years. Hence, barring chance coincidences, detected cosmic rays will not point back to known astrophysical transients [25] . However, detected UHECRs should point back (within the errors from deflection) to the host galaxies. As type Ibc SNe occur mostly in HI-rich spirals, the detected correlation with HI-selected galaxies [34] is consistent with our hypothesis. Similarly, direct detection of UHECRs from say SN 2009bb is unlikely. However, photo–hadron interaction between accelerated protons or nuclei and optical photons from the underlying SN may produce pions, which then decay ( or ) to give high-energy neutrinos [38] , [39] . Neutrinos have no electric charge, hence, they are not deflected by the intergalactic magnetic fields. They have very low rest masses compared with their very high energies and will travel at nearly the speed of light. These neutrinos will not be temporally coincident with the initial core collapse as the number of accelerated charged particles, which are the source of neutrinos grows with time. The peak of the high-energy neutrino flux will approximately coincide with the peak in bolometric luminosity (at around a week after explosion for SN 2009bb) as the most number of photons will be available for interaction with the accelerated hadrons. Hence, high-energy neutrinos may by found in future by neutrino detectors like the IceCube, in directional and rough temporal coincidence with relativistic SNe. How to cite this article: Chakraborti S. et al . Ultra-high-energy cosmic ray acceleration in engine-driven relativistic supernovae. Nat. Commun. 2:175 doi: 10.1038/ncomms1178 (2011).